Capture and conversion of CO2at ambient conditions by a conjugated microporous polymer Conjugated microporous polymers are a new class of porous materials with an extended π-conjugation in an amorphous organic framework. Owing to the wide-ranging flexibility in the choice and design of components and the available control of pore parameters, these polymers can be tailored for use in various applications, such as gas storage, electronics and catalysis. Here we report a class of cobalt/aluminium-coordinated conjugated microporous polymers that exhibit outstanding CO 2 capture and conversion performance at atmospheric pressure and room temperature. These polymers can store CO 2 with adsorption capacities comparable to metal-organic frameworks. The cobalt-coordinated conjugated microporous polymers can also simultaneously function as heterogeneous catalysts for the reaction of CO 2 and propylene oxide at atmospheric pressure and room temperature, wherein the polymers demonstrate better efficiency than a homogeneous salen-cobalt catalyst. By combining the functions of gas storage and catalysts, this strategy provides a direction for cost-effective CO 2 reduction processes. CO 2 emissions are a serious problem in the establishment of a sustainable society and are driving the implementation of green chemistry concepts. These emissions are widely considered to be a primary factor in global climate change [1] , [2] . The development of efficient and cost-effective methods for CO 2 capture and sequestration is an important goal for human society over the course of this century. To replace the currently employed industrial method of chemical sorption of CO 2 , which has high energy demands, researchers have developed processes by which CO 2 is adsorbed over zeolite, carbon, alumina and metal-organic frameworks (MOFs) [3] , [4] . It has also been proposed that captured CO 2 be deposited in underground reservoirs [5] . However, as it is the most environmentally abundant C1 building block available, the chemical conversion of captured CO 2 to high-value products is attractive [6] . One such product is the cyclic carbonate formed during the coupling of CO 2 and epoxides, which has wide applications in the pharmaceutical and fine chemical industries. Although the formation of cyclic carbonate via homogeneous catalysts has been industrialized, the process requires high temperatures and pressures, and product separation is difficult. The development of a heterogeneous catalyst for synthesizing cyclic carbonate at mild conditions remains a challenge [7] , [8] , [9] . The combination of CO 2 capture and conversion is an attractive strategy for efficiently reducing CO 2 emissions. It is essential that the materials used in this strategy be able to capture and convert CO 2 at atmospheric pressure and room temperature with only heat from the surrounding environment to avoid the generation of new CO 2 . Thus far, no material has been identified that satisfies these requirements. Conjugated microporous polymers (CMPs) are of great interest because their porous structures contain organic functionalities that, in principle, allow significant synthetic diversification. A variety of CMPs have been developed for applications in areas such as gas sorption [10] , [11] , molecular separation [12] , electronics [13] and catalysis [14] , [15] . More recently, several demonstrations of use of metal-functionalized CMPs that combine valuable chemical and physical properties, such as both gas sorption and catalytic activities, have been reported. For example, a Li atom-doped CMP that we developed displayed very high H 2 sorption because the lithium ion, formed by electron transfer between the lithium atom and its support, functions as an active centre for the absorption of molecular hydrogen [16] . Chen et al . [17] have reported a metalloporphyrin-derived CMP with high catalytic activity for the oxidation of thiols. The Cooper group has developed two strategies for synthesizing metal-organic CMPs with high catalytic activities [15] . These materials combine the physical properties and porous structures of the conjugated framework backbones of CMPs with the chemical properties of the incorporated metal-organic moieties. Similar incorporation of metal-organic moieties in CMPs may lead to materials capable of both CO 2 capture and its simultaneous conversion. In this study, we demonstrate a class of metal-functionalized CMPs synthesized with Salen-Co/Al complexes and 1,3,5-triethynylbenzene. These new Salen-Co/Al–coordinated CMPs (hereafter referred to as Co-CMPs and Al-CMPs) were capable of capturing and converting CO 2 at room temperature and atmospheric pressure. The Salen-Co/Al complex has previously been identified as a homogenous catalyst in the formation of cyclic carbonate from CO 2 and epoxides at relatively low temperatures and pressures [18] , [19] , [20] , [21] , and the conjugated porous frameworks of CMPs have been proven as appropriate candidates for the capture of CO 2 (ref. 22 ). Our combination of these two components led to CMPs that satisfy the requirements for the cost-effective reduction of CO 2 . Synthetic procedure To prepare Co-CMP, we first synthesized the dibromo-functionalized precursor monomers (Salen-Co) by a complexation reaction of cobalt acetate (Co(OAc) 2 ) and (R,R)- N ′ N ′-bis(5-bromo-3-tert-butyl-salicylidene)-1,2-cyclohexanediaminate (Salen) [23] . After purification, the resultant precursors were treated with 1,3,5-triethynylbenzene in the presence of a Pd(0) catalyst in toluene under reflux to produce CMPs (Co-CMP) ( Fig. 1 , Method A). Al-CMP was prepared using a different method ( Fig. 1 , Method B), the synthesis details of which are given in the Supplementary Methods . The Co-CMP structure, modelled computationally, had a porous three-dimensional network structure arising from its three-pronged linkages ( Fig. 2a ). The resultant polymers, Co-CMP and Al-CMP, were chemically stable, completely insoluble in organic solvents, and exhibited high thermal stabilities ( T dec >300 °C, see Supplementary Fig. S1 ). 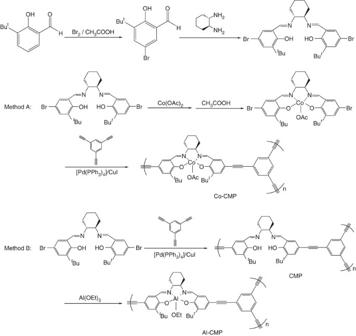Figure 1: Synthesis of Co-CMP (Method A) and Al-CMP (Method B). Full experimental details and characterization are provided in theSupplementary Methods. Figure 1: Synthesis of Co-CMP (Method A) and Al-CMP (Method B). Full experimental details and characterization are provided in the Supplementary Methods . 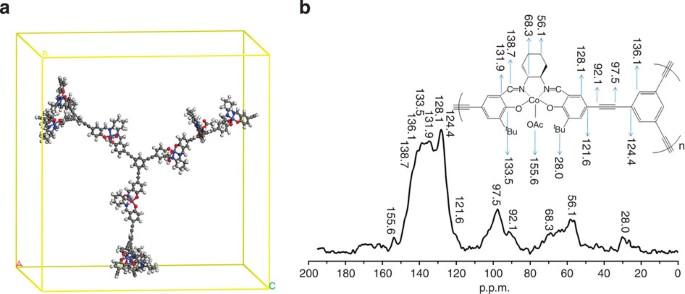Figure 2: Computer-modelled structure and NMR spectrum of Co-CMP. (a) Three-dimensional view of Co-CMP in an amorphous periodic cell. (b) Solid-state1H–13C CP/MAS NMR spectrum of Co-CMP recorded at a spinning speed of 10 kHz. Full size image Figure 2: Computer-modelled structure and NMR spectrum of Co-CMP. ( a ) Three-dimensional view of Co-CMP in an amorphous periodic cell. ( b ) Solid-state 1 H– 13 C CP/MAS NMR spectrum of Co-CMP recorded at a spinning speed of 10 kHz. Full size image Structural characterization The molecular structure of Co-CMP was assessed with 1 H– 13 C CP/MAS solid-state nuclear magnetic resonance (NMR), as shown in Fig. 2b . The resonance assignment was confirmed by the 1 H– 13 C CP/MAS kinetics. The peaks at 95.7 and 92.1 p.p.m. were ascribed to sp-hybridized –C≡C– atoms, and the shoulder at 155.6 p.p.m. was assigned to –C=O groups in the carboxylate. The peaks at 121.6, 124.4, 128.1, 131.9, 133.5 and 136.1 p.p.m. corresponded to the carbon atoms of the aromatic rings in the polymer, and the peak at 138.7 p.p.m. was ascribed to carbons in the –C=N groups. The peaks at 56.1 and 68.3 p.p.m. were ascribed to sp 2 -hybridized –CH 2 carbons and sp-hybridized –CH carbons in the cyclohexyl moiety. The lowest intensity peak at 28.0 p.p.m. was ascribed to the –CH 3 groups. Al-CMP was characterized using 1 H– 13 C cross-polarization magic-angle spinning (CP/MAS) NMR spectroscopy ( Supplementary Fig. S2a ). With the exception of the carbonyl groups (–C=O), the resonances of Al-CMP were similar to those observed in Co-CMP. The morphological structures of Co-CMP and Al-CMP are shown in Fig. 3 . The scanning electron microscope (SEM) pictures ( Fig. 3a ) show that Co-CMP and Al-CMP consist of relatively uniform solid sub-micron spheres. The majority of the mesopores in the polymers can be ascribed to the interparticulate porosity that exists between the agglomerated primary microgel particles. The high-resolution transmission electron microscope images of Co-CMP and Al-CMP ( Fig. 3b ) show the presence of nanometre-sized pores (~0.5 nm sizes) on the polymer surface. According to these images (additional images are given in Supplementary Fig. S3 ), the polymers were wholly featureless at the length scales observed. 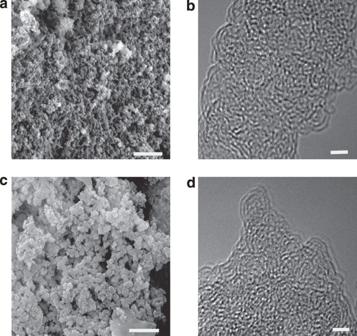Figure 3: Morphological structures of Co-CMP and Al-CMP. SEM images of the microporous conjugated polymers Co-CMP (a) and Al-CMP (c) (scale bar, 500 nm). High-resolution transmission electron microscope (HR-TEM) images of Co-CMP (b) and Al-CMP (d) (scale bar, 2 nm). Figure 3: Morphological structures of Co-CMP and Al-CMP. SEM images of the microporous conjugated polymers Co-CMP ( a ) and Al-CMP ( c ) (scale bar, 500 nm). High-resolution transmission electron microscope (HR-TEM) images of Co-CMP ( b ) and Al-CMP ( d ) (scale bar, 2 nm). Full size image CO 2 adsorption capacity The porous properties of the polymers were investigated by nitrogen adsorption analyses at 77.3 K ( Fig. 4a ) and CO 2 adsorption analyses at 298 K ( Fig. 4b and Supplementary Fig. S4 ). All of the polymers showed type I nitrogen gas sorption isotherms according to the IUPAC classifications, indicating that the metallated polymers consisted of both micropores and mesopores. No significant change in the pore size distribution was observed between Co-CMP and Al-CMP ( Supplementary Fig. S5 ). According to the size distribution curves calculated by NLDFT, the median value of the pore size in the polymers is 0.5 nm. 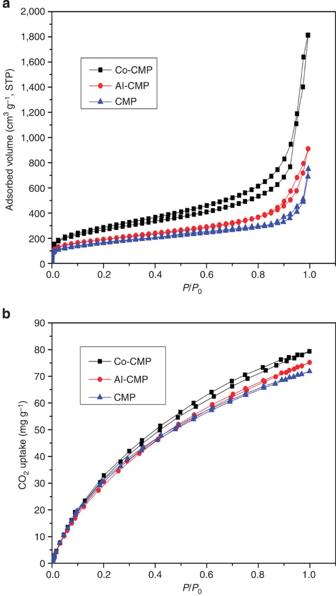Figure 4: Gas uptake data for conjugated microporous polymers. (a) N2adsorption and desorption isotherms for CMP (blue triangles), Co-CMP (black squares) and Al-CMP (red circles) at 77.3 K. (b) CO2sorption and desorption isotherms for CMP (blue triangles), Co-CMP (black squares) and Al-CMP (red circles) at 298 K. Figure 4: Gas uptake data for conjugated microporous polymers. ( a ) N 2 adsorption and desorption isotherms for CMP (blue triangles), Co-CMP (black squares) and Al-CMP (red circles) at 77.3 K. ( b ) CO 2 sorption and desorption isotherms for CMP (blue triangles), Co-CMP (black squares) and Al-CMP (red circles) at 298 K. Full size image Other porosity properties, such as the CO 2 adsorption capacity, Brunauer–Emmett–Teller (BET) surface area and pore volume are summarized in Table 1 . Co-CMP had a much higher BET surface area (965 m 2 g −1 ) than either Al-CMP (798 m 2 g −1 ) or CMP (772 m 2 g −1 ). According to Table 1 , the total pore volume of Co-CMP was 2.81 cm 3 g −1 , which is substantially larger than the volume of several high-pore-volume MOFs, including UMCM-2 (2.31 cm 3 g −1 ) (ref. 24 ), MOF-177 (1.89 cm 3 g −1 ) (ref. 25 ) and NOTT-112 (1.62 cm 3 g −1 ) (ref. 26 ). Cobalt and aluminium were detected in the polymers using inductively coupled plasma-optical emission spectroscopy (ICP–OES). Metal contents in the polymers were found to be 7.19 wt.% Co and 3.46 wt.% Al, respectively, which are slightly less than the theoretical values of 8.20 wt.% Co and 4.01 wt.% Al. SEM/EDX analyses ( Supplementary Fig. S6 ) showed that the Co/N ratio in Co-CMP and the Al/N ratio in Al-CMP were 1:2.9 and 1:2.5, respectively, indicating that a small portion of the Salen units in the CMPs were not coordinated to metal atoms. Table 1 Physical properties for conjugated microporous polymers. Full size table The CO 2 sorption properties of the polymers were investigated using volumetric methods at 298 K ( Table 1 ). The CO 2 adsorption isotherms of both Co-CMP and Al-CMP displayed reversible adsorption capacity ( Fig. 4b and Supplementary Fig. S4 ). When the pressure P (actual pressure) approached 760 mm Hg (that is, P / P 0 approached 1), the CO 2 uptake reached 79.3 mg g −1 and 76.5 mg g −1 in Co-CMP and Al-CMP, respectively. Under the same conditions, CMP absorbed 71.0 mg g −1 CO 2 , possibly as a result of the relatively low BET surface area. We compared the CO 2 adsorption capacities of Co-CMP and Al-CMP with those of the MOFs in the literature. Under identical conditions to those in our study, CO 2 uptakes of 106.7 mg g −1 , 71.5 mg g −1 and 10.4 mg g −1 were reported for MC-BIF-2H, MC-BIF-3H and MC-BIF-5H [27] , respectively. Despite having a relatively low surface area, Co-CMP and Al-CMP exhibited comparatively high CO 2 absorption, indicating that Co-CMP and Al-CMP are good CO 2 capture materials. Catalytic activity We utilized Co-CMP and Al-CMP as solid catalysts for CO 2 transformation. Co-CMP and Al-CMP show exceptional catalytic activity in the conversion of propylene oxide (PO) to propylene carbonate (PC) under mild experimental conditions ( Table 2 ). Entries 1–7 in Table 2 show the performances of various catalytic systems at atmospheric pressure and room temperature. As shown in entry 1, the homogeneous Salen-Co-OAc catalyst afforded the coupling reaction with a 77.1% yield under standard conditions. In the absence of co-catalyst nBu 4 NBr (TBAB), the PO/CO 2 coupling reaction catalysed by Co-CMP yields only 6.7% PC after 48 h ( Table 2 , entry 2). Moreover, in the absence of Co-CMP, the coupling reaction catalysed by the co-catalyst TBAB (ref. 28 ) alone gave a 20.4% yield. However, catalysts that combined Co-CMP with a co-catalyst TBAB promoted the coupling reaction with an 81.5% yield at room temperature and atmospheric pressure ( Table 2 , entry 4). This is notably better than the 77.1% yield already described for the homogeneous catalyst Salen-Co-OAc. Enrichment of CO 2 concentrations near the catalytic centres located in the pore structures of the CO 2 -capturing heterogeneous catalyst likely explains enhanced performance of Co-CMP compared with Salen-Co-OAc. Al-CMP also exhibited excellent catalytic activity under the same experimental conditions and catalysed the coupling reaction with a yield of 78.2% ( Table 2 , entry 5). We also compared the catalytic performances of Co/Al-CMP with the catalysts currently used in industry for PO/CO 2 coupling, such as KI and KI/β-CD [29] . At atmospheric pressure and room temperature, KI and KI/β-CD exhibited poor catalytic activities with yields of 3.8% and 3.9%, respectively (entry 6 and 7). The plot in Fig. 5a relates yield (PC) to reaction time at atmospheric pressure and room temperature. The ranking of catalytic activities from largest to smallest is Co-CMP>Al-CMP> Salen-Co-OAc >>TBAB>KI/β-CD≈KI. To the best of our knowledge, Co-CMP and Al-CMP are the only heterogeneous catalysts that can catalyse the PO/CO 2 coupling reaction at atmospheric pressure and room temperature [21] . Table 2 Influence of experimental conditions on propylene carbonate yields. 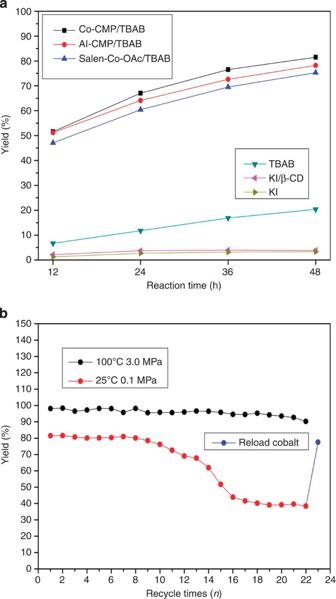Figure 5: The catalytic activity of various catalytic systems and the recycling of Co-CMP. (a) The yield (PC) depending on reaction time at atmospheric pressure and room temperature. (b) The recycling stability of Co-CMP under various experimental conditions. * Full size table Figure 5: The catalytic activity of various catalytic systems and the recycling of Co-CMP. ( a ) The yield (PC) depending on reaction time at atmospheric pressure and room temperature. ( b ) The recycling stability of Co-CMP under various experimental conditions. Full size image To further demonstrate the superiority of the heterogeneous Co/Al-CMP catalysts, we carried out reactions with various catalytic systems (entries 8–15, Table 2 ) at relatively high temperatures (100 °C) and CO 2 pressures (3.0 MPa). When the reaction was catalysed by the homogeneous catalyst Salen-Co-OAc (entry 8, Table 2 ), the PC yield was 84.6%. By using Co-CMP and Al-CMP as catalysts, the PC yields were increased to 98.1% and 91.2%, respectively (entries 10 and 11, Table 2 ). In the absence of Co-CMP or Al-CMP, the PC yield was only 31.0% with TBAB as catalyst under the same conditions ( Table 2 , entry 9). Entries 12 and 13 indicate that oxygen and water in the reaction systems had little effect on the PC yields catalysed by Co-CMP. However, the addition of a small amount of water (0.2 ml) dramatically decreased the PC yields catalysed by Al-CMP (entry 14). We also compared the catalytic performances of Co/Al-CMP with the industrial catalysts (KI and KI/β-CD) at elevated temperature and pressure. The catalytic activities of KI and KI/β-CD are shown in entries 15 and 16 in Table 2 . The comparison clearly indicates that even under these conditions Co-CMP (98.1%) and Al-CMP (91.2%) had superior catalytic activities to that of KI (3.0%) and KI/β-CD (13.2%) in the conversion of PO into PC. Co-CMP also proved effective in large-scale catalysis by experiments run over 60 h at 3.5 MPa CO 2 and 130 °C, producing a PO turn over number (TON) of 40,660 ( Supplementary Fig. S7 ). To investigate the recycling stability of Co-CMP and Al-CMP, experiments were repeated with a large number of iterations. We found that Co-CMP could be reused up to 22 times without any significant changes under high CO 2 pressure (3 MPa) and elevated temperature (100 °C) ( Fig. 5b ). At room temperature and atmospheric pressure, the reaction yield dropped slightly from 81.5% to 70.6% after 11 runs and dramatically dropped to 38.4% after 22 runs (1,056 h reaction time), as shown in Fig. 5b . The cobalt content in Co-CMP after 1,056 h reaction time was determined to be 0.89 wt.% by ICP–OES. This indicated that the cobalt had a degree of solubility in the reaction system. Cobalt can be reloaded onto Co-CMP by refluxing Co-CMP (120 mg) and Co(OAc) 2 (80 mg) in anhydrous tetrahydrofuran (12 ml) for 24 h. The reloaded Co-CMP completely recovered its catalytic activity ( Fig. 5b , blue circle). Unfortunately, the recycling stability of Al-CMP was much worse. Reaction yields dropped from 78.2% to 51.3% after only three times (see Supplementary Fig. S8 ), perhaps as a result of the highly hygroscopic nature of Salen-Al in Al-CMP. Trace water in the system may form inactive Al species and kill reactivity. This explanation is consistent with the observation in entry 14 of Table 2 . The exceptional catalytic performances of the Co-CMP and Al-CMP catalysts were consistent with a mechanism in which the metallic moiety on the polymer was instrumental in the activation of reactant species ( Supplementary Fig. S9 ). The ring opening of PO by a quaternary ammonium salt TBAB resulted in a cobalt- or aluminium-bound alkoxide in an S N 2-type reaction. At the same time, CO 2 coordinated to the same metal ion and allowed intermolecular transfer of the alkoxide to coordinated CO 2 , resulting in a metal carbonate capable of cyclization to form PC with regeneration of the catalysts [18] . Quantum calculations were used to investigate this mechanism. All of the calculated intermediates and transition states are listed in the Supplementary Tables S1–S8 . The catalytic centre (Co-(Salen)) was clipped from Co-CMP. As shown in Supplementary Fig. S10 , the reaction mechanism was presumed to occur in four steps, starting from the reaction of PO with the catalyst (Co-(Salen)), which was found to be exothermic (Δ E =−7.56 kcal mol −1 ) and barrier-free. This was assumed to be a relatively spontaneous process. The next step was the attack of the nucleophile (Br − ) on PO, which was considered the most difficult step in the reaction as it had the largest activation energy (Δ E # =8.89 kcal mol −1 ). The third step was the insertion of CO 2 , which was assumed to be a simple intramolecular process rather than a rate-determining step. The activation energy (ΔE # ) was 0.72 kcal mol −1 , and the reaction energy Δ E was −3.24 kcal mol −1 . The last step was the formation of the PC, but as this reaction was exothermic (ΔE=−9.46 kcal mol −1 ) with a ΔE # of 4.70 kcal mol −1 , it was concluded that this step occurred easily. This last step was a backbiting reaction; the nucleophile (Br - ) left the product as the product simultaneously desorbed from the catalyst. These four steps are exothermic with small activation energies; therefore, we assumed that the reaction could occur without additional energy input. In conclusion, the polymers Co-CMP and Al-CMP, both of which have high BET surface areas, displayed excellent CO 2 adsorption capacities. Furthermore, when co-catalysed with a quaternary ammonium salt TBAB, Co-CMP and Al-CMP displayed exceptionally high catalytic activities in the conversion of PO and CO 2 to PC at atmospheric pressure and room temperature. A single catalyst (Co-CMP) could be reused up to 22 times without a significant decrease in catalytic activity. These findings provide a new direction for the simultaneous capture and conversion of CO 2 . Materials synthesis All of the reactions and manipulations were carried out under argon with the use of standard inert atmosphere and Schlenk techniques or inside a nitrogen-filled glovebox. Detailed procedures for the ligand synthesis are reported in the Supplementary Methods . We synthesized Co-CMP via the Pd(0)-catalysed cross-coupling of 1,3,5-triethynylbenzene with [(R,R)- N ′ N ′-bis(5-bromo-3 -tert-butyl-salicylidene)-1,2-cyclohexanediaminate] cobalt (III) acetate. Al-CMP was prepared using a different method. We first prepared a CMP by Sonogashira–Hagihara cross-coupling of 1,3,5-triethynylbenzene and [(R,R)- N ′ N ′-bis(5-bromo-3-tert-butyl-salicylidene)-1,2-cyclohexane diaminate] in the presence of Pd(0) as a catalyst. This polycondensation reaction resulted in a series of porous networks that incorporated metal-binding sites. After purification and drying, the precursor CMP was treated with Al(OEt) 3 in toluene under reflux to obtain the polymer Al-CMP. Synthesis of Co-CMP Salen-Co-OAc (400 mg, 0.57 mmol), 1,3,5-triethynylbenzene (180 mg, 1.2 mmol), CuI (50 mg) and tetrakis-(triphenylphosphine) palladium(0) (100 mg) were dissolved in a mixture of toluene (15 ml) and triethylamine (6 ml). The reaction mixture was heated to 40 °C and stirred for 1 h under an argon atmosphere (to exclude oxygen and prevent any homocoupling of the alkyne monomers). Next, the reaction mixture was heated to 80 °C, stirred for 72 h and then cooled to room temperature. The insoluble precipitated polymer was filtered and washed four times with dichloromethane, methanol, water and acetone to remove any unreacted monomers or catalyst residues. Further purification of the polymer was carried out by Soxhlet extraction with methanol and dichloromethane (volume ratio=1:1) for 48 h. The product was dried in a vacuum for 24 h at 70 °C and isolated as a brown powder (yield: 460 mg, 79.3%). Synthesis of CMP 1,3,5-Triethynylbenzene (300 mg, 2 mmol), Salen (296 mg, 0.5 mmol), CuI (80 mg) and tetrakis-(triphenylphosphine) palladium-(0) (120 mg) were dissolved in a mixture of toluene (10 ml) and Et 3 N (5 ml). The reaction mixture was heated to 40 °C and stirred for 1 h under an argon atmosphere (to exclude oxygen and prevent any homocoupling of the alkyne monomers). Next, the reaction mixture was heated to 85 °C, stirred for 72 h and then cooled to room temperature. The insoluble precipitated polymer was filtered and washed four times with dichloromethane, methanol, water and acetone to remove any unreacted monomers or catalyst residues. Further purification of the polymer was carried out by Soxhlet extraction with water, dichloromethane, acetone and methanol (volume ratio=1:1:1:1) for 24 h. The product was dried in a vacuum for 24 h at 70 °C and isolated as a brown powder (yield: 481 mg, 80.8%). Synthesis of Al-CMP CMP (150 mg) was added to a solution of Al(OEt) 3 (300 mg) in 30 ml of toluene, and the suspension was then refluxed for 24 h. The mixture was cooled to room temperature, and the insoluble precipitated network polymer was filtered and washed four times with dichloromethane, water, methanol and acetone to remove the unreacted aluminium complex. Further purification of the polymer was carried out using a Soxhlet extraction with water, acetone, dichloromethane and methanol for 24 h. The product was then dried under vacuum for 24 h at 70 °C to yield 280 mg of brown powder (Al-CMP) (yield: 280 mg, 62.2%). Synthesis of PC A pre-dried 50-ml autoclave was charged with Co-CMP (or Al-CMP) (50–100 mg) and PO (1.75 ml, 25 mmol) in the atmosphere. Next, the assembled autoclave was purged of air three times with CO 2 . After the CO 2 (3.0 MPa) was introduced, the reaction mixture was stirred at 100 °C for 1 h. The autoclave was cooled to room temperature, and the CO 2 was released. The reaction mixture was then dissolved with ethyl acetate (30 ml), and the insoluble solid material was filtered. Removing the solvent from the filtrate yielded a pale yellow oil substance. Further purification of the crude product was carried out by column chromatography (yield: 90–99.6%). How to cite this article: Xie, Y. et al . Capture and conversion of CO 2 at ambient conditions by a conjugated microporous polymer. Nat. Commun. 4:1960 doi: 10.1038/ncomms2960 (2013).